Electroreductive hydroxy fluorosulfonylation of alkenes An electroreductive strategy for radical hydroxyl fluorosulfonylation of alkenes with sulfuryl chlorofluoride and molecular oxygen from air is described. This mild protocol displays excellent functional group compatibility, broad scope, and good scalability, providing convenient access to diverse β-hydroxy sulfonyl fluorides. These β-hydroxy sulfonyl fluoride products can be further converted to valuable aliphatic sulfonyl fluorides, β-keto sulfonyl fluorides, and β-alkenyl sulfonyl fluorides. Further, some of these products showed excellent inhibitory activity against Botrytis cinerea or Bursaphelenchus xylophilus , which could be useful for potent agrochemical discovery. Preliminary mechanistic studies indicate that this transformation is achieved through rapid O 2 interception by the alkyl radical and subsequent reduction of the peroxy radical, which outcompete other side reactions such as chlorine atom transfer, hydrogen atom transfer, and Russell fragmentation. Sulfonyl fluorides have found wide applications in chemical biology [1] , [2] , materials science [3] , [4] , organic synthesis [5] , [6] , and other areas in chemistry [7] , [8] , since sulfur(VI) fluoride exchange (SuFEx) reactions were recognized as a new generation of click reaction in 2014 [9] . In this context, a range of key methods have been developed for the construction of FSO 2 -containing molecules [5] , [7] , [8] , [9] , primarily including aryl sulfonyl fluorides [10] , [11] , [12] , [13] , alkenylsulfonyl fluorides [14] , [15] , [16] , alkynylsulfonyl fluorides [17] , and β-keto sulfonyl fluorides [18] , [19] , [20] . On the other hand, alcohols are one of the most ubiquitous functional groups in natural products and bioactive molecules. The incorporation of a hydroxyl group can significantly change the binding affinity and pharmacokinetic properties of drug molecules [21] , [22] , [23] . As such, we envisioned that the combined β-hydroxy sulfonyl fluoride motif might exhibit improved bioactivity compared to previously reported β-keto sulfonyl fluorides (Fig. 1a , I) [19] . Fig. 1: Context of the work. a Retrosynthetic analysis. b Reduction of β-keto sulfonyl fluorides. c Challenges for hydroxyl fuorosulfonylation of alkenes. d Electroreductive hydroxy fluorosulfonylation of alkenes. Full size image Radical difunctionalization of alkenes would be an ideal strategy for the construction of β-hydroxy sulfonyl fluoride scaffolds (Fig. 1a ., II), as it could allow the simultaneous introduction of HO and FSO 2 functionalities onto prevalent alkene feedstocks. Moreover, the direct reduction of the ketone group in β-keto sulfonyl fluorides failed to afford β-hydroxy sulfonyl fluorides in our hands (Fig. 1b ). While several elegant protocols for the radical fluorosulfonylation [24] , [25] , [26] , [27] , [28] , [29] , [30] and radical hydroxysulfonylation [31] , [32] , [33] have been developed, 1,2-hydroxy fluorosulfonylation of alkenes remains a synthetic challenge and FSO 2 radical precursors are strictly limited so far (Fig. 1a ). Recently, Liao discovered that radical Int-1 abstracted Cl-atom too fast to be trapped with other reagents, and alkenylsulfonyl fluorides were formed from the radical fluorosulfonylation of olefins (Fig. 1c ) [29] . Later, the same group avoided the fast Cl-atom transfer process with a benzimidazolium-based sulfonyl fluoride reagent as the radical precursor, enabling the trapping of benzylic carbocation with simple alcohols (Fig. 1c ) [27] . Both Studer [28] and Glorius [24] groups introduce bifunctional reagents for the radical olefin 1,2-difunctionalization, providing β-alkynyl sulfonyl fluorides and β-imino sulfonyl fluoride, respectively. Despite these advances, synthetic access to β-hydroxy sulfonyl fluorides has not been reported to date. Electrochemistry has emerged as a sustainable tool in organic chemistry [34] , [35] , [36] , [37] , [38] , [39] , which in many cases is complementary to photoredox catalysis [40] . Indeed, the electrochemical oxidation has been extensively applied for the difunctionalization of alkenes [41] , [42] , [43] , [44] . However, the electroreductive strategy [45] , [46] , [47] , [48] , [49] , [50] for the alkene difunctionalizations is substantially less explored. It is noteworthy that an electroreductive radical-polar crossover strategy for the difunctionalization of alkenes has recently been disclosed by Lin [51] . Afterward, several methods for difunctionalization of alkenes were developed rapidly via electroreductive chemistry [52] , [53] , [54] . We herein report the successful development of an electroreductive 1,2-hydroxyl fluorosulfonylation of alkenes, which produces diverse β-hydroxy sulfonyl fluorides (Fig. 1d ). Taking advantage of feasible access to FSO 2 • at a very low reduction potential (FSO 2 Cl, E p/2 = 0.45 V vs SCE, see Supplementary Fig. 11 ), we could avoid the further reduction of alkyl radical intermediate (i.e., benzyl radical, E p/2 = −1.6 V vs SCE) [51] . The consumption of FSO 2 Cl at the cathode results in a low local concentration of FSO 2 Cl. Thus, a rapid O 2 interception by the alkyl radical would outcompete the Cl-atom transfer from the low concentration of FSO 2 Cl. Identification of a suitable reduction system would be key to suppressing the competing pathway including Russell fragmentation [55] , [56] , hydrogen atom transfer (HAT) [26] , and carbon anion generation. Furthermore, the synthetic utilities have been demonstrated by versatile follow-up derivatizations and biological activity studies. Reaction development In our initial survey, we investigated the designed 1,2-hydroxyl fluorosulfonylation toward 3 by employing our previous conditions for electrochemical oxo-fluorosulfonylation of phenylacetylene (Fig. 2a ) [19] . However, the reaction of styrene ( 1a ) and FSO 2 Cl ( 2 ) provided the desired β-hydroxy sulfonyl fluoride 3 in only 10% yield, along with 13% yield of β-keto sulfonyl fluoride 4 and a complex mixture of other inseparable products (Fig. 2b ). This result clearly indicates that Russell fragmentation of alkyl peroxy radical may compete with the desired reduction pathway [55] , [56] . Fig. 2: Initial studies for hydroxy fluorosulfonylation. a Our previous work. b Initial trials for the synthesis of β-hydroxy sulfonyl fluoride 3 . 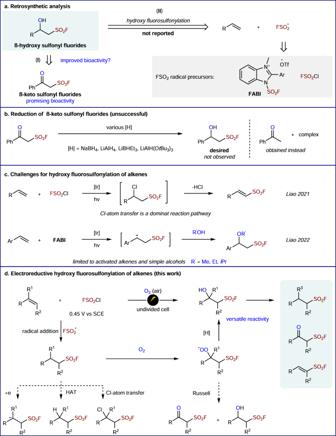Fig. 1: Context of the work. aRetrosynthetic analysis.bReduction of β-keto sulfonyl fluorides.cChallenges for hydroxyl fuorosulfonylation of alkenes.dElectroreductive hydroxy fluorosulfonylation of alkenes. Full size image Next, we explored the reaction conditions with styrene ( 1a ) and FSO 2 Cl ( 2 ) in an undivided cell equipped with an aluminum plate anode and a zinc plate cathode under air at room temperature (Table 1 ). When constant current conditions were employed, the potential gradually increased over the reaction time, and more byproducts were formed. As such, constant cell voltage conditions were employed to avoid undesired redox processes. Inspired by Mukaiyama hydration [57] , [58] , various hydride donors were examined to suppress ketone formation. After extensive optimization, we were pleased to find that with Et 3 SiH (2.0 equiv) and B 2 (OH) 4 (2.5 equiv) using LiClO 4 as the electrolyte in Et 2 O (0.016 M) under 8 V constant cell voltage conditions, the desired olefin difunctionalization product 3 was isolated in 96% yield (entry 1). Without Et 3 SiH and B 2 (OH) 4 , only 40% yield of 3 was obtained along with other inseparable byproducts (entry 2). Control experiments showed that Et 3 SiH and B 2 (OH) 4 both were important (entries 3&4). Other silanes were screened but resulted in lower reaction efficiency (entries 5–7). The difunctionalization reaction did not proceed when using radical initiator Et 3 B or reducing reagent BH 3 ·THF instead of B 2 (OH) 4 (entry 8). These results indicated that B 2 (OH) 4 was not likely employed as a radical initiator or simple borane precursor. Lewis acids BF 3 ·Et 2 O and B(C 6 F 5 ) 3 led to decreased yields (entries 9 and 10). Since B 2 (OH) 4 could be used as a deoxygenating agent [59] and boronic acids were able to reduce peroxides [60] , here B 2 (OH) 4 likely acted as a reducing agent for the reduction of the hydroperoxide intermediate. It is known that the electrode material can significantly influence electron transfer [61] . The choice of electrodes is critical for the success of this transformation, although it is empirical. Much lower yields were observed using other electrodes, such as Zn(+)/Al(−) and Al(+)/Al(−) (entries 11 and 12), while no product was detected using Zn(+)/Zn(−) and C(+)/C(−) (entry 13). Specifically, a cathode material with higher overpotential is typically preferred to suppress the undesired proton reduction [61] . Interestingly, a non-sacrificial anode with graphite felt (GF) was also effective in providing 3 in 75% yield (entry 14). Evaluation of different solvents uncovered that this reaction only proceeds in ethereal solvents such as Et 2 O (entry 1), THF (entry 15), and 1,4-dioxane (entry 16). The desired transformation was completely suppressed when swapping to non-ethereal solvents (entry 17). Additionally, increasing or decreasing the concentration turned out to be less effective (entries 18 and 19). Finally, we demonstrated the essential role of oxygen in the air by performing the reaction under nitrogen atmosphere in which styrene 1 was fully recovered (entry 20). This observation can be rationalized by the fact that β-fragmentation of the FSO 2 • is feasible [28] , [62] , thus reversibly leading to the starting material styrene without enough radical trapping reagent at the cathode (e.g., O 2 and FSO 2 Cl). Surprisingly, reaction without electricity also furnished the desired product 3 in 78% yield (entry 21). Presumably, an electron donor–acceptor (EDA) complex was formed between styrene 1a and FSO 2 Cl [63] , [64] , thus leading to the generation of FSO 2 • upon daylight irradiation (see Supplementary Fig. 16 ). However, this EDA strategy exhibited an extremely limited styrene scope (see Supplementary Fig. 15 ). Table 1 Optimization of the reaction conditions a Full size table Substrate scope With the optimized conditions in hand, we next evaluated the substrate scope of this electroreductive hydroxy fluorosulfonylation with respect to styrenes (Fig. 3a ). Pleasingly, 2-, 3-, or 4-halogenated styrenes (Br, Cl, F) were well tolerated, furnishing the desired products 5 – 9 in 43–78% yield. Styrenes bearing electron-withdrawing groups (-CF 3 , -CHO, -CO 2 Me, -NO 2 , -CN) and electron-donating groups (-Me, -OMe, -OAc, -OTs) were viable substrates, delivering β-hydroxy sulfonyl fluorides 10 – 21 in moderate to excellent yields. In particular, the aldehyde functionality could not be reduced under our conditions and the desired product 11 was isolated in 56%. Moreover, the sterically hindered 2,4,6-trimethylstyrene reacted to afford difunctionalization product 18 in 49% yield. In addition, substrates bearing biphenyl, naphthyl, and benzothiophene reacted under standard conditions, furnishing the corresponding products 22 – 25 in 40–59% yield. Of note, α-methylstyrene and α-bromostyrene were successfully converted to the desired products 26 and 27 in 62% and 20% yield, respectively. Estrone and cholestanol derivatives 28 and 29 were isolated in 36% and 55% yield, respectively. Fig. 3: Substrate scope. a Scope of styrenes. b Scope of terminal alkenes. c Scope of internal alkenes. d Site-selective hydroxyl-fluorosulfonylation. a conditions: 1 (0.2 mmol), 2 (2 equiv), Et 3 SiH (2 equiv), B 2 (OH) 4 (2.5 equiv), LiClO 4 (0.1 M), Et 2 O (0.016 M), aluminum anode (10 mm × 15 mm × 1 mm), zinc cathode (10 mm × 15 mm × 1 mm), cell voltage ( U cell = 8 V), undivided cell, air, rt, 16 h. Isolated yield. BRSM based on recovered starting material. b 2 mmol scale. Full size image Besides styrenes, unactivated terminal alkenes were also evaluated in this hydroxy fluorosulfonylation (Fig. 3b ). Terminal olefins with different long chains and branched chains were employed, giving β-hydroxy sulfonyl fluorides 30 – 34 in 40–65% yield. A variety of functional groups, including ketone, ester, carboxylic acid, pentylphosphonates, and bromide, were compatible under our conditions, leading to 35 – 40 in 33–74% yield. We examined the scope of internal alkenes next (Fig. 3c ). An arrange of FSO 2 -functionalized cycloalkanols could be accessed under mild conditions, including cyclopentanol ( 41 ), cyclohexanol ( 42 ), 1-indanol ( 43 ), and tetrahydronaphthalenol ( 44 ) from cyclic alkenes. Trisubstituted olefins such as 3-methylindene, 2-methylindene, and 4-methyl-1,2-dihydronaphthalene were transformed to sulfonyl fluorides 45 – 47 in 51–66% yield. Acyclic olefins such as β-methylstyrene or cinnamyl acetate were also effective, providing 48 and 49 in moderate yields. Site-selective functionalization of dienes could be realized under reaction conditions (Fig. 3d ). As expected, ( E )-2-methyl-1-phenyl-1,3-butadiene and γ-terpinene were selectively functionalized at the less steric olefin, leading to sulfonyl fluorides 50 and 51 . Interestingly, 1,7-octadiene and 1,4-cyclohexadiene could also selectively furnish β-hydroxy sulfonyl fluorides 52 and 53 while retaining one olefin group. In vitro biological activities . We also evaluated the promising bioactivities of these sulfonyl fluorides. 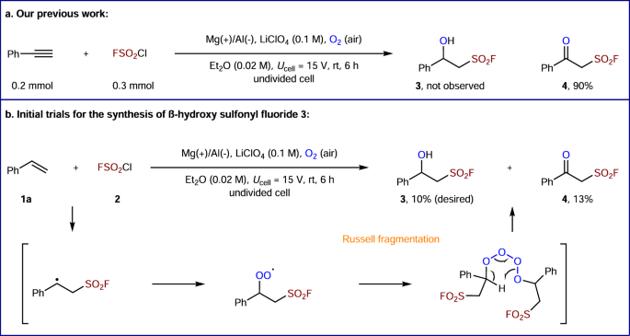Fig. 2: Initial studies for hydroxy fluorosulfonylation. aOur previous work.bInitial trials for the synthesis of β-hydroxy sulfonyl fluoride3. As shown in Table 2 , compounds 22, 23, 37 , and 45 displayed good antifungal activities against Botrytis cinerea , which is a serious pathogenic fungus causing severe damage to plant species worldwide [65] . Notably, 45 displayed strong inhibitory activity with EC 50 of 2.67 μg/mL, which was obviously better than chlorothalonil (see Supplementary Table 11 and Supplementary Figs. 18 – 20 ). Furthermore, several compounds exhibited significant nematicidal activity ( 35 , LC 50 = 25.92 μg/mL) against Bursaphelenchus xylophilus , which is a serious threat to pine trees and causes severe damage to forest ecosystems (see Supplementary Tables 14 and 15 ) [66] , [67] . Of note, these β-hydroxy sulfonyl fluorides typically showed improved bioactivities than β-keto sulfonyl fluorides from our previous work (see Supplementary Tables 13 and 16 ). Table 2 In vitro antifungal activities against Botrytis cinerea a Full size table Representative derivatizations The synthetic utility of the hydroxyl fluorosulfonylation was further demonstrated (Fig. 4 ). Firstly, the electrolysis of 8 mmol of 1a with 2 was performed under standard conditions, and the desired product 3 was obtained in 95% yield (1.55 g). Then, the alcohol moiety in β-hydroxy sulfonyl fluoride 3 could be converted efficiently to acetate or trimethyl silyl ether, resulting in 54 or 55 . In addition, oxidation of the alcohol group delivered β-keto sulfonyl fluoride 4 in 87% yield. In the presence of AlCl 3 , 2-phenyl-2-(thiophen-2-yl) ethanesulfonyl fluoride 56 could be obtained by a Friedel–Crafts reaction of 3 with thiophene. Finally, dehydration of the alcohol in 3 was promoted by AlCl 3 to deliver ( E )-2-phenylethene-1-sulfonyl fluoride 57 . Fig. 4: Representative derivatizations. DCE 1,2-dichloroethane, DBU diazabicycloundecene. For details, please see Supplementary Information (SI) . Full size image Mechanistic studies Several mechanistic experiments were conducted to gain further insight into the mechanism of this electroreductive hydroxyl fluorosulfonylation (Fig. 5a ). First, a radical process was possible based on the observation that TEMPO or BHT completely inhibits the reaction. FSO 2 radical was also trapped by 1,1-diphenylethylene 58 with the isolation of 59 in 10% yield. Next, subjecting the observed byproduct 4 to our standard conditions did not lead to the desired product 3 , supporting that they were formed via a divergent pathway. Moreover, constant potential experiments indicated that the cathodic potential of our standard reaction was lower than −0.1 V, and a higher reductive potential led to lower reaction efficiency (Fig. 5b ). Furthermore, cyclic voltammetry studies showed that Et 3 SiH or B 2 (OH) 4 were not involved into the electrochemical process (see Supplementary Figs. 12 and 13 ). Fig. 5: Mechanistic experiments and proposal. a Mechanistic studies. b Constant potential electrolysis. c Proposed mechanism. Full size image Finally, a plausible reaction pathway for this electroreductive process is outlined in Fig. 5c , based on the abovementioned studies and our previous reports [18] , [19] . The reaction starts from the generation of FSO 2 radical via cathodic reduction of FSO 2 Cl. Thus, the concentration of FSO 2 Cl in the cathode surface region is much lower than that of styrene 1a and O 2 . This unique feature of electrosynthesis may facilitate the reaction of benzylic radical intermediate I , produced from the radical addition of FSO 2 • to 1a , preferentially with O 2 to afford benzyl peroxy radical II . Thus, the chlorine atom transfer with FSO 2 Cl can be suppressed, in contrast to previous work via photocatalysis. Subsequently, a HAT between Et 3 SiH and II delivers hydroperoxide III , which can be reduced by B 2 (OH) 4 via intermediate IV to form borate VI [59] , [60] , alone with B(OH) 3 detected by 11 B NMR analysis. Hydrolysis of VI produces the desired product 3 . Meanwhile, halogen atom transfer (XAT) of the triethylsilyl radical with FSO 2 Cl regenerates the FSO 2 radical. The constant voltage is required to improve the efficiency of this radical chain process because Et 3 Si• can undergo homocoupling to form hexaethyldisilane, which is confirmed by HRMS-ESI analysis. Other competing reaction pathways are also possible (Fig. 5c , right), particularly in the absence of Et 3 SiH and B 2 (OH) 4 . In summary, we have realized an electroreductive hydroxyl fluorosulfonylation of alkenes that proceeds through a rapid O 2 interception by the alkyl radical and subsequent reduction of the peroxy radical. The protocol tolerates many functional groups, furnishing diverse β-hydroxy sulfonyl fluorides with potential applications for agrochemical development from alkenes under mild conditions. Furthermore, versatile follow-up derivatizations have showcased the synthetic utility to access valuable aliphatic sulfonyl fluorides, β-keto sulfonyl fluorides, and β-alkynyl sulfonyl fluorides. General procedure for the synthesis of 3 A 20-mL vial with one aluminum (anode) plate electrode (10 mm × 15 mm × 1 mm), one zinc (cathode) plate electrode (10 mm × 15 mm × 1 mm) and a stir bar was charged with LiClO 4 (130 mg, 0.1 M), Et 2 O (12 mL, 0.016 M), B 2 (OH) 4 (0.5 mmol, 2.5 equiv), Et 3 SiH (0.4 mmol, 2 equiv) and 1a alkenes (0.2 mmol). 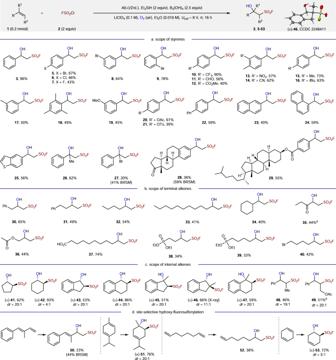Fig. 3: Substrate scope. aScope of styrenes.bScope of terminal alkenes.cScope of internal alkenes.dSite-selective hydroxyl-fluorosulfonylation.aconditions:1(0.2 mmol),2(2 equiv), Et3SiH (2 equiv), B2(OH)4(2.5 equiv), LiClO4(0.1 M), Et2O (0.016 M), aluminum anode (10 mm × 15 mm × 1 mm), zinc cathode (10 mm × 15 mm × 1 mm), cell voltage (Ucell= 8 V), undivided cell, air, rt, 16 h. Isolated yield. BRSM based on recovered starting material.b2 mmol scale. Then, ClSO 2 F was added (0.4 mmol, 2 eq, 1 M in anhydrous PhCF 3 ). The mixture was electrolyzed at a constant cell voltage of 8 V for 16 h under an atmosphere of air (1 atm, balloon). 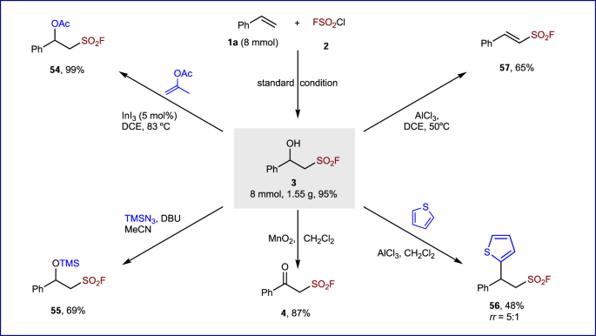Fig. 4: Representative derivatizations. DCE 1,2-dichloroethane, DBU diazabicycloundecene. For details, please seeSupplementary Information (SI). 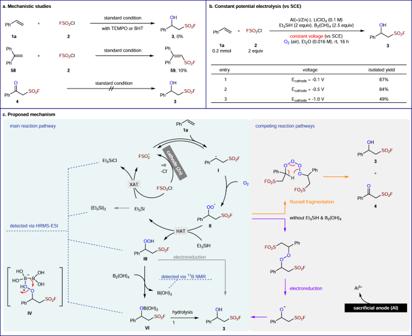Fig. 5: Mechanistic experiments and proposal. aMechanistic studies.bConstant potential electrolysis.cProposed mechanism. Subsequently, the reaction was quenched with water, and electrodes were rinsed with EtOAc. The resulting mixture was extracted with EtOAc and the combined organic layers were dried over Na 2 SO 4 and concentrated in vacuo. The residue was purified by column chromatography to afford the desired product 3 (PE/DCM/EA = 20/20/1 ~ 5/5/1).